An asymmetric heterodomain interface stabilizes a response regulator–DNA complex Two-component signal transduction systems consist of pairs of histidine kinases and response regulators, which mediate adaptive responses to environmental cues. Most activated response regulators regulate transcription by binding tightly to promoter DNA via a phosphorylation-triggered inactive-to-active transition. The molecular basis for formation of stable response regulator–DNA complexes that precede the assembly of RNA polymerases is unclear. Here, we present structures of DNA complexed with the response regulator KdpE, a member of the OmpR/PhoB family. The distinctively asymmetric complex in an active-like conformation reveals a unique intramolecular interface between the receiver domain (RD) and the DNA-binding domain (DBD) of only one of the two response regulators in the complex. Structure–function studies show that this RD–DBD interface is necessary to form stable complexes that support gene expression. The conservation of sequence and structure suggests that these findings extend to a large group of response regulators that act as transcription factors. In constantly changing environments, the ability of bacteria to survive, grow and colonize various niches depends on adaptive responses controlled by two-component signal transduction systems (TCSs) [1] , [2] . TCSs are absent in metazoans, but present in archaea, lower eukaryotes and plants and are especially abundant in bacteria [3] . Therefore, they are attractive targets for drug development to control infections and antibiotic resistance. There are an average of 25 TCSs per bacterium [4] making them significant players in environmental sensing. TCSs control a wide variety of processes, including quorum sensing, osmoregulation, nutrient uptake, sporulation, redox response, stress response, nitrogen fixation, virulence, antibiotic resistance and chemotaxis [1] , [5] , [6] . Most TCSs consist of a membrane-bound sensor histidine kinase with a variable sensing domain attached to a conserved cytoplasmic kinase domain. In this elegant signalling circuit, stimuli perceived by the histidine kinase are relayed by phospho-transfer reactions to response regulators (RRs), which instigate cellular responses [5] , [7] . RRs have a conserved receiver domain (RD) and a variable output domain [6] , [8] , [9] . More than 60% of output domains bind DNA to act as transcription factors [10] . Termination of signalling occurs through dephosphorylation of the RR by auto hydrolysis, histidine kinase-mediated dephosphorylation [11] and by auxiliary phosphatases [12] , [13] . RRs are molecular switches that exist in equilibrium between inactive and active states [14] , [15] . The population shifts to an active state on phosphorylation of an invariant aspartate in the RD [7] , [16] . The activated RD regulates the activity of the linked output domain. The current paradigm for phosphorylation-induced regulation in RRs invokes use of interfaces created between surfaces of domains rather than large conformational transitions within individual domains (reviewed by Gao and Stock [17] ). One well-described surface, defined by the α4-β5-α5 secondary structure elements of the RD was identified in both activating and inhibitory processes [18] , [19] . In some RRs, the α4-β5-α5 surface of RDs in an inactive conformation sequesters the DNA-binding domain (DBD) to occlude interaction with DNA [20] , [21] . Phosphorylation leads to the formation of a two-fold symmetrical dimer formed by the α4-β5-α5 surface, thus the inhibition is relieved [22] , [23] . In other RRs, no inhibition of DNA binding is observed (for example, OmpR). Nevertheless, the affinity of RRs to DNA is always higher when the RD is phosphorylated [24] , [25] . The specific interactions that stabilize the high-affinity complexes between activated RRs and DNA remains unknown due to lack of structure of any full-length RR–DNA complex. KdpE is a member of the OmpR/PhoB family, the largest group of RRs identified in bacteria. The KdpD/KdpE signalling circuit is activated when the histidine kinase KdpD senses a drop in external K + concentration or an upshift in ionic osmolarity, resulting in the expression of a heterooligomeric transporter KdpFABC [26] . KdpFABC pumps K + , the major osmolyte to restore cellular homeostasis [27] , [28] . KdpE also regulates colonization and virulence genes: in Staphylococcus aureus , a major agent of drug-resistant infections [29] , [30] and in enteropathogenic bacteria via QseC/KdpE pathway [31] , [32] . In this study, we present structures of full-length KdpE bound to its cognate DNA. The KdpE molecules in an active-like conformation create a previously unrecognized asymmetric inter-domain interface between the RD and DBD of one of the two KdpE molecules in the complex. Structure–function studies show the importance of this asymmetric interface in the regulation of gene expression. Our findings suggest that the molecular basis for the formation of stable, high-affinity complexes capable of promoting transcription depends on the formation of multiple interfaces between surfaces of domains of KdpE molecules. Characterization of the RR–DNA complex The aspartyl phosphate moiety formed during RR phosphorylation is unstable; the reported half-life is minutes to a few hours [33] . Therefore, RRs in the activated state are studied either as complexes with the phosphoryl-mimic beryllium fluoride (BeF 3 − ) (ref. 34 ) or by using mutants that were constitutively active [35] , [36] , [37] , [38] . Attempts to prepare activated KdpE by incubation with phosphomimetics failed due to protein precipitation; a similar observation was reported for the isolated RD of KdpE [23] . Alternatively, an approach successfully used to produce constitutively active phenotype in other RRs by replacing the active-site aspartate with a glutamate was attempted by changing aspartate 52 of KdpE to a glutamate. The KdpE-D52E variant was incapable of gene expression under permissive conditions ( Fig. 1a ). We identified an active variant KdpE-E216A with residue change in the DBD that exhibits higher levels of reporter β-galactosidase production independent of the external K + concentration ( Fig. 1a ). The phenotype of KdpE-E216A could be due to changes in protein conformation or due to hyperphosphorylation. A double-substitution E216A/D52A lacking Asp 52, the site of KdpE phosphorylation was capable of reporter β-galactosidase production, indicating that gene expression was independent of phosphorylation state of the RD. Purified KdpE-E216A bound to a DNA molecule containing the recognition sites (half-sites S1 and S2 (ref. 39 )) with ninefold greater affinity than did KdpE ( Fig. 1b ). Surface plasmon resonance (SPR) analysis was conducted by injecting KdpE and KdpE-E216A over a DNA-bound chip ( Fig. 1c,d ). Data from three independent replicates were used to estimate the off-rate and the s.e.m. The off-rate of KdpE-E216A (0.006±0.001 s −1 ) was slower than that of KdpE (0.016±0.003 s −1 ) indicating formation of a more stable DNA complex by KdpE-E216A. RRs of the OmpR/PhoB family bind to DNA more tightly in an activated state [24] , [25] . The data on KdpE-E216A suggest that it mimics some of the properties that would be expected of KdpE in an activated (phosphorylated) state. 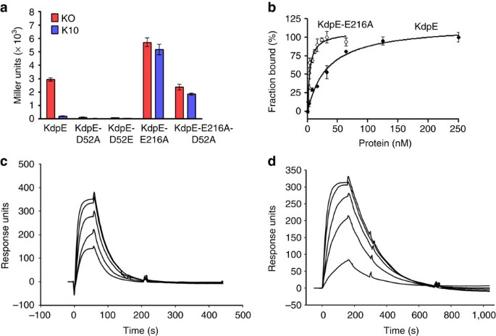Figure 1: Characterization of the RR KdpE and its variants. (a) β-Galactosidase expression inE. colicells co-expressing histidine kinase KdpD with wild-type KdpE, KdpE-E216A, double substituent KdpE-E216A-D52A or inactive KdpE-D52A and KdpE-D52E in inducing media without K+(red squares) or in 10 mM K+(blue squares). (b) Analysis of binding of KdpE (black circles) and KdpE-E216A (white circles) to DNA by fluorescence anisotropy; estimated dissociation constants were 30±4.0 nM and 3.5±0.5 nM, respectively. Error bars represent s.e.m. of three independent measurements. (c,d) SPR analysis. The binding to DNA immobilized on a chip was analyzed by injecting various concentrations of (c) KdpE (50–300 nM) and (d) KdpE-E216A (10–50 nM). Figure 1: Characterization of the RR KdpE and its variants. ( a ) β-Galactosidase expression in E. coli cells co-expressing histidine kinase KdpD with wild-type KdpE, KdpE-E216A, double substituent KdpE-E216A-D52A or inactive KdpE-D52A and KdpE-D52E in inducing media without K + (red squares) or in 10 mM K + (blue squares). ( b ) Analysis of binding of KdpE (black circles) and KdpE-E216A (white circles) to DNA by fluorescence anisotropy; estimated dissociation constants were 30±4.0 nM and 3.5±0.5 nM, respectively. Error bars represent s.e.m. of three independent measurements. ( c , d ) SPR analysis. The binding to DNA immobilized on a chip was analyzed by injecting various concentrations of ( c ) KdpE (50–300 nM) and ( d ) KdpE-E216A (10–50 nM). Full size image Structures of KdpE–DNA and KdpE-E216A–DNA complexes To determine the structure of full-length RR–DNA complexes, crystallization trials were conducted with KdpE and KdpE-E216A complexed to double-stranded DNA of varied lengths with either blunt ends or overhangs of one or two bases. Crystallization trials were successful only with DNA molecules 30 bp in length with blunt ends for both KdpE–DNA and KdpE-E216A–DNA complexes. In this DNA molecule, the two half-sites S1 and S2 are separated by five bases and have extensions of four and nine bases, respectively, on either side of the half-sites. The crystallographic details of the KdpE–DNA and KdpE-E216A–DNA complexes at 2.95 Å and 2.53 Å, respectively, are shown in Table 1 . The higher resolution of data from the KdpE-E216A–DNA complex allowed modelling of all 30 bp of DNA, whereas in the KdpE–DNA only 24 bp were modelled ( Fig. 2 ; Supplementary Figs 1 and 2 ). The structures of both complexes are essentially the same with overall root mean square deviations (r.m.s.d.) of 0.324 Å ( Supplementary Table 1 ). Table 1 Crystallographic data and refinement statistics. 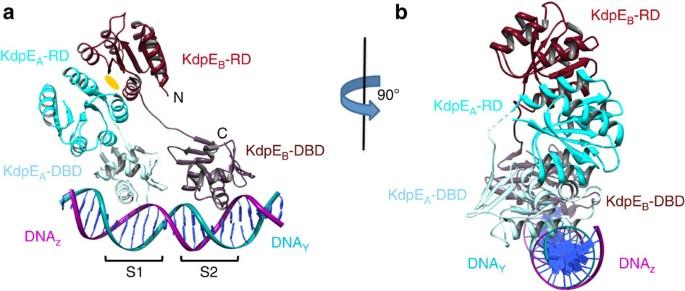Figure 2: Structure of KdpE–DNA complex. (a,b) Ribbon representation of two copies of KdpE complexed to its cognate DNA viewed perpendicular and parallel to the helical axis of DNA. Chains KdpEAand KdpEBRDs are coloured cyan and maroon, respectively, whereas the DBDs are shaded in light blue and brown, respectively. The DNA chains Y and Z are coloured blue and pink. S1 and S2 are the half-sites that form the recognition sites on DNA. The oval in yellow indicates the two-fold symmetry axis for the RDs. The linker region connecting RD and DBD of chain KdpEBwas modelled, whereas three residues missing in KdpEAare indicated by a dotted line. Full size table Figure 2: Structure of KdpE–DNA complex. ( a , b ) Ribbon representation of two copies of KdpE complexed to its cognate DNA viewed perpendicular and parallel to the helical axis of DNA. Chains KdpE A and KdpE B RDs are coloured cyan and maroon, respectively, whereas the DBDs are shaded in light blue and brown, respectively. The DNA chains Y and Z are coloured blue and pink. S1 and S2 are the half-sites that form the recognition sites on DNA. The oval in yellow indicates the two-fold symmetry axis for the RDs. The linker region connecting RD and DBD of chain KdpE B was modelled, whereas three residues missing in KdpE A are indicated by a dotted line. Full size image The overall structure of the KdpE–DNA complex is skewed, positioning the RDs away from the −35 region of the promoter, the binding site for the RNA polymerase ( Fig. 2 ). In this complex, the two KdpE molecules, namely KdpE A and KdpE B , are bound to DNA half-sites S1 and S2 respectively. Each KdpE protomer consists of an RD (residues 1–120) and a DBD (residues 129–225) connected by a linker. We refer to KdpE A and KdpE B as compact and extended subunits, respectively, to indicate the direct interaction between RD and DBD in KdpE A and lack thereof of such interactions in KdpE B . The linker conformations in the two KdpE molecules differ, because the compact subunit (KdpE A ) forms a RD–DBD interface, whereas the extended molecule (KdpE B ) lacks such interactions between the equivalent domains. The KdpE–DNA complex is asymmetric due to two features ( Fig. 2 ). First, the two RDs form a symmetrical dimer, but the associated DBDs are positioned on DNA asymmetrically with respect to each other, because they bind to the S1 and S2 half-sites that are 6-bp direct repeat sequences [39] ( Fig. 2a ). Second, the half-sites are separated by 5-bp sequences, which position the two KdpE molecules on one side of the B-DNA helix ( Fig. 2b ). Conformation of the RDs All RRs have an architecturally conserved RD that undergoes limited structural changes during the inactive-to-active state transition. Structures of phosphomimetic-complexed RDs have been compared with the non-phosphorylated counterparts to define the activated state conformation. This state involves the repositioning of side chains of two switch residues (Ser/Thr and Tyr) from an outward-facing conformation in the inactive state to a position proximal to and facing the active site on phosphorylation [40] , [41] , [42] as well as the formation of a symmetrical RD-RD dimer involving α4-β5-α5 faces [18] . In both the KdpE–DNA ( Fig. 3a ) and KdpE-E216A–DNA complexes ( Supplementary Fig. 3 ), the conserved switch residues S79 and Y98 are in the inward facing conformation, and the α4-β5-α5 surfaces of the RDs form symmetrical dimers. Based on the above criteria, the RDs in the KdpE–DNA and KdpE-E216A–DNA complexes in the absence of phosphomimetics appear to have a conformation similar to that of other activated RDs. A similar (active) conformation was reported by the Stock group for the RD of KdpE (PDB ID 1ZH2) in the absence of phosphoryl analogues [23] . RDs achieving an active-state conformation in the absence of phosphoryl analogues possess what is referred to as an ‘active-like’ state (as per Bachhawat and Stock [43] ). 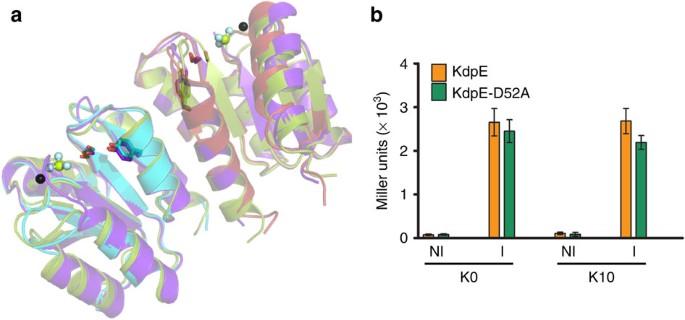Figure 3: Conformation of RDs of KdpE and the effect of protein overproduction on gene expression. (a) Comparison of structures of various RDs of KdpE. The structure of RDs from KdpE–DNA complex was superposed on the structures of RDs of KdpE complexed with BeF3−(PDB ID: 1ZH4 (ref.23)) and the RD of the inactive variant KdpE-D52A. The colouring scheme used is: cyan and pink for the RDs from chains A and B, respectively, in the KdpE–DNA complex structure (this study), green RD from 1ZH4 and purple for RD from KdpE-D52A structure (this study). The switch residues Ser79 and Tyr98 of KdpE are shown in stick representation. The single black sphere and bonded multiple spheres represent magnesium ion and BeF3−, respectively, are from 1ZH4. The overlaid structures emphasize that the RDs in KdpE–DNA complex and of the inactive variant, KdpE-D52A are in an active-like conformation despite the absence of phosphomimetics and similar to the conformation of RD of KdpE bound to BeF3−. (b) Effect of RR concentration on reporter gene expression. KdpE and non-phosphorylatable variant KdpE-D52A were expressed inE. coliRH003 (lacking KdpE and KdpD) in media without K+(K0) and in 10 mM K+(K10). The levels of RRs were manipulated by having no inducer (NI) or by addition of 1.0 mM IPTG (I) resulting in low (basal) and high levels of RR expression, respectively. β-galactosidase activity was reported as Miller units for three independent measurements with error bars representing s.e.m. Figure 3: Conformation of RDs of KdpE and the effect of protein overproduction on gene expression. ( a ) Comparison of structures of various RDs of KdpE. The structure of RDs from KdpE–DNA complex was superposed on the structures of RDs of KdpE complexed with BeF 3 − (PDB ID: 1ZH4 (ref. 23 )) and the RD of the inactive variant KdpE-D52A. The colouring scheme used is: cyan and pink for the RDs from chains A and B, respectively, in the KdpE–DNA complex structure (this study), green RD from 1ZH4 and purple for RD from KdpE-D52A structure (this study). The switch residues Ser79 and Tyr98 of KdpE are shown in stick representation. The single black sphere and bonded multiple spheres represent magnesium ion and BeF 3 − , respectively, are from 1ZH4. The overlaid structures emphasize that the RDs in KdpE–DNA complex and of the inactive variant, KdpE-D52A are in an active-like conformation despite the absence of phosphomimetics and similar to the conformation of RD of KdpE bound to BeF 3 − . ( b ) Effect of RR concentration on reporter gene expression. KdpE and non-phosphorylatable variant KdpE-D52A were expressed in E. coli RH003 (lacking KdpE and KdpD) in media without K + (K0) and in 10 mM K + (K10). The levels of RRs were manipulated by having no inducer (NI) or by addition of 1.0 mM IPTG (I) resulting in low (basal) and high levels of RR expression, respectively. β-galactosidase activity was reported as Miller units for three independent measurements with error bars representing s.e.m. Full size image To capture the RD in an inactive conformation, we expressed, purified and crystallized the isolated RD of the non-phosphorylatable variant KdpE-D52A. The structure determined using SAD phasing at 2.2 Å ( Table 1 ) shows a two-fold dimer with switch residues facing inside, that is, an active-like conformation ( Fig. 3a ). Of note, the crystallization conditions, the space groups and the crystal packing are different for: the RD of KdpE [23] , the RD of KdpE-D52A and the RDs in the KdpE and KdpE-E216A complexed to DNA. The effect of high protein concentrations (found in crystals) on inactive-to-active state transitions was evaluated by overexpressing KdpE and the non-phosphorylatable variant KdpE-D52A in RH003 cells in the absence of the histidine kinase KdpD. β-galactosidase production under non-permissive (10 mM) and permissive concentrations (0 mM) of K + were measured. Cells producing low levels of KdpE grown under conditions permissive to reporter expression show little β-galactosidase activity due to lack of histidine kinase ( Fig. 3b ). Levels of β-galactosidase production achieved when KdpE or KdpE-D52A was overexpressed ( Fig. 3b ) was comparable to co-expression of KdpE and KdpD ( Fig. 1a ). These data suggest high concentrations of KdpE and KdpE with D52A substitution are capable of driving gene expression in the absence of phosphorylation by forcing an inactive- to active-like conformational transition. Intramolecular RD–DBD interface of the compact subunit The RD–DBD interface of the compact subunit is characterized by specific polar contacts between side chains and buries a relatively small surface area of 375 Å 2 per monomer. Residues from helix α3 and the loop connecting α3 and β4 of the RD form a web of interactions that involve water molecules and side chains of DBD residues. Two sets of interactions between the DBD and the RD are observed. The first set ( Fig. 4a ) involves a 3.27 Å salt bridge between the carboxylate of D66 of the RD and R158 of the DBD. The residues are also bridged by a water molecule that is located 2.45 Å and 2.67 Å from residues D66 and R158, respectively. The guanidinium group of R158 hydrogen bonds with three water molecules that are central players in this network of interactions. The water molecules form hydrogen bonds to each other and to the indole group of W70 of the RD and the side chain of R141 on β8 of the DBD. This set of interactions is bookended by an interaction between R141 and W70 at the carboxyl-terminal end of helix α3 of the RD. The residue R141 is unique, because it participates in two interfaces: in RD–DBD interactions in the compact subunit and in the DBD–DBD interface between molecules. On the other side of the compact subunit, a second set of interactions ( Supplementary Fig. 4 ) involve the side-chain and the main-chain carbonyl oxygen of Q69 of RD and the side chains of N165 and Q179 situated on helices α7 and α8 of the DBD, respectively. These interactions are further stabilized by hydrogen bonds between water and the carbonyl oxygen of Q69 and the side chain of N165 from the DBD. 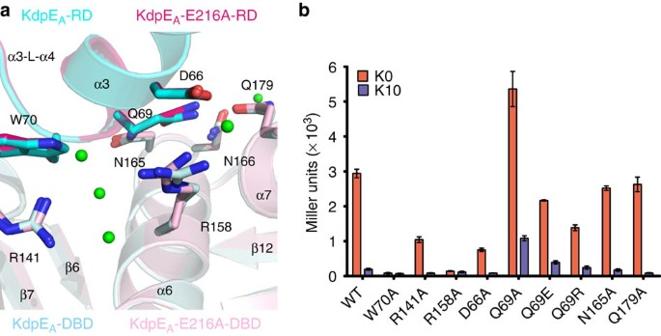Figure 4: Intramolecular heterodomain interactions. (a) Interface between RD and DBD of the compact subunit KdpEAand KdpEA-E216A. Side chains involved in polar interactions are shown as sticks. α3-L-α4 denotes the loop between α-helices 3 and 4, and green spheres represent water molecules (from the KdpEA-E216A–DNA structure). (b) Effects of mutations on reporter β-galactosidase production expressed as Miller units in media without K+and in 10 mM K+conditions, which are permissive and non-permissive for gene expression, respectively. Error bars represent s.e.m. of three independent measurements. Figure 4: Intramolecular heterodomain interactions. ( a ) Interface between RD and DBD of the compact subunit KdpE A and KdpE A -E216A. Side chains involved in polar interactions are shown as sticks. α3-L-α4 denotes the loop between α-helices 3 and 4, and green spheres represent water molecules (from the KdpE A -E216A–DNA structure). ( b ) Effects of mutations on reporter β-galactosidase production expressed as Miller units in media without K + and in 10 mM K + conditions, which are permissive and non-permissive for gene expression, respectively. Error bars represent s.e.m. of three independent measurements. Full size image The specific interactions at the RD–DBD interface of the compact molecule, and the overall structural asymmetry in the complex led us to hypothesize that the observed RD–DBD interface of the compact subunit is essential for the formation of a stable, active RR–DNA complex. The hypothesis makes a testable prediction that mutations disrupting the RD–DBD interface will affect protein function. Indeed, changes in any of the four residues involved in the first set of interactions (D66 and W70 in the RD and R141 and R158 in the DBD) to alanine significantly reduced or eliminated reporter gene expression under K + -limiting conditions ( Fig. 4a,b ). The replacement of residues involved in the second set of interactions between the RD and the DBD ( Supplementary Fig. 4 ) by alanine had little effect on gene expression except for the residue Q69 at the tip of helix α3 of RD. The Q69A substitution resulted in increased β-galactosidase production at the repressive and inductive K + concentrations. The replacement of Q69 with the isosteric residue E or with a positively charged residue R resulted in wild-type-like β-galactosidase production. The structure–function analysis suggests that a specific set of residues, D66, Q69, W70, R141 and R158, at the RD–DBD interface plays an important role in activation of gene expression at the permissive concentration of K + . Role of the intermolecular DBD–DBD interface In structures of KdpE–DNA and KdpE-E216A–DNA complexes, the DBD–DBD interface buries a modest 350 Å 2 of solvent accessible surface per monomer ( Fig. 5a ; Supplementary Fig. 5 ). Therefore, the stability of the DBD–DBD interface depends on DBDs binding to adjacent DNA half-sites and on the formation of the larger RD-RD dimer interface that will increase the local concentration of DBDs, thereby stabilizing the complex. Superposition of our previously reported structure of an isolated DBD of KdpE [39] onto the KdpE-E216A–DNA complex revealed small changes in conformations of Cα positions between DNA-bound and -free states of the DBD ( Supplementary Table 1 , Supplementary Fig. 6a ). A notable difference is a flip in the side chain of H151 towards the DNA in the DNA-complexed forms, which brings Nε2 of H151 to within 2.8 Å of OP1 of dT14 of the DNA. A similar flip in H151 towards DNA is also observed in wild-type KdpE–DNA complex structure ( Supplementary Fig. 6b ). 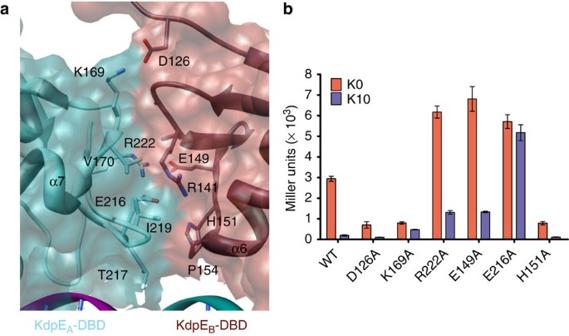Figure 5: Intermolecular DBD–DBD interactions. (a) Interface between a pair of DBDs bound to direct repeats on DNA. Side chains involved in interactions are shown as sticks. (b) Effects of mutations of interfacial residues on β-galactosidase production expressed as Miller units in media without K+(K0) and in 10 mM K+(K10) conditions permissive and non-permissive for gene expression, respectively. Error bars represent s.e.m. of three independent measurements. Figure 5: Intermolecular DBD–DBD interactions. ( a ) Interface between a pair of DBDs bound to direct repeats on DNA. Side chains involved in interactions are shown as sticks. ( b ) Effects of mutations of interfacial residues on β-galactosidase production expressed as Miller units in media without K + (K0) and in 10 mM K + (K10) conditions permissive and non-permissive for gene expression, respectively. Error bars represent s.e.m. of three independent measurements. Full size image In the structure of KdpE-E216A–DNA complex, the E216A substitution maps to the asymmetric intermolecular interface between the DBDs ( Supplementary Fig. 5 ). In the wild-type structure, the residue E216 forms a weak interaction with H141 (4.2 Å between OE1 of E216 and ND1 of H151) of the adjacent subunit, whereas it forms a strong salt bridge (2.5 Å) with NH1 of R222 of the same subunit ( Fig. 5a ). E216 is part of a network of interactions involving R222, E149, H144, D126 and K169 ( Fig. 5a ), therefore the effect of these residues on gene expression was evaluated. Replacements to alanine that disrupt salt-bridges and hydrogen bonds at the interface resulted in variants that respond differently to K + levels in the test medium ( Fig. 5b ). In case of substitutions situated at the periphery of the interface, such as H151A, D126A and K169A, the levels of β-galactosidase production are lower, but they still respond to changes in the K + concentrations. However, changes to the residues buried deeper in the interface (R222A, E149A and E216A) have elevated levels of reporter gene expression both under permissive and non-permissive conditions. None of the changes to residues disrupted DNA binding ( Supplementary Fig. 7 ) or brought about significant alterations in the level of protein expression ( Supplementary Fig. 8 ). Because these substitutions continue to respond to changes in K + concentrations, they are likely to have altered threshold for activation. The altered threshold may arise as a result of changes to the surface of KdpE adjacent to the RNA polymerase affecting its interactions with RNA polymerase or due to the effects of substitutions on the KdpE–DNA complex stability. Our data support the latter possibility: one of the E149A mutations map to a surface of one of the DBD (KdpE B -DBD) that is buried in the DBD–DBD interface and other is on the surface of a DBD (KdpE A -DBD) that is situated away from the RNA polymerase-binding site on the promoter. Although the mechanism for altered threshold of activation by KdpE-E216A is not clear, our studies reveal that the relatively small DBD–DBD interface is highly sensitive to amino-acid substitutions resulting in either higher or lower levels of gene expression that depends on position of the altered residue. Interaction of DBDs with DNA The carboxyl-terminal winged helix-turn-helix motif of the DBD positions helix α8 into the major groove of DNA ( Fig. 6a ). This permits base-specific interactions allowing specific binding at DNA half-sites. The two DNA-bound DBDs have similar conformations to each other and to the isolated DBD of KdpE [39] ( Table 1 ), suggesting the lack of significant conformational changes on binding DNA. However, distinct differences in interactions with DNA are seen: At the S1 half-site, four side chains of KdpE A -DBD interact with four bases, whereas all six bases of S2 are contacted by the DBD of KdpE B via 11 hydrogen bonds ( Fig. 6b ). The differential binding of KdpE is unrelated to the single base pair difference between half-site S1 (TTTATA) and S2 (TTTACA). Previously, we showed that the variable base has no effect on binding of the isolated DBD of KdpE to DNA and that the binding at each half-site occurs with equal affinity and no detectable cooperativity [39] . The differences in interaction at S1 and S2 half-sites probably arise from the difference in orientation of the two DBDs with respect to DNA. KdpE B -DBD at site S2 is rotated by 36 degrees compared with DBD at site S1. 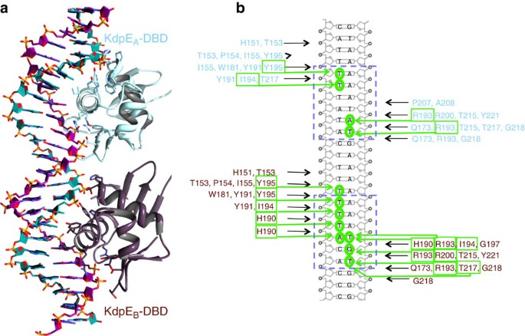Figure 6: DNA–protein interactions. (a) Interaction of DBDs of chains KdpEAand KdpEBwith major grooves at half-sites S1 and S2, respectively. The colouring scheme is as inFig. 2. Side chains that interact with nucleotide bases are shown in stick representation. (b) Contact map illustrating residues within 4.0 Å distance from nucleotide bases (green arrows) and the DNA backbone (black arrows). The half-sites S1 and S2 are boxed. Figure 6: DNA–protein interactions. ( a ) Interaction of DBDs of chains KdpE A and KdpE B with major grooves at half-sites S1 and S2, respectively. The colouring scheme is as in Fig. 2 . Side chains that interact with nucleotide bases are shown in stick representation. ( b ) Contact map illustrating residues within 4.0 Å distance from nucleotide bases (green arrows) and the DNA backbone (black arrows). The half-sites S1 and S2 are boxed. Full size image Conformational changes resulting from the activation of RDs are well studied [17] . The first change is within the RD, and the second includes the association between RDs. Others, particularly changes in an RR–DNA complex involving heterodomain interactions are poorly described. The first structure of an intact RR complexed to DNA that is distinctly asymmetric provides insights into the formation of a stable RR–DNA complex by identifying a new RD–DBD interface formed by only one of the two RRs in the complex. The first two changes in activated RDs involve reorientation of side chain of switch residues of the RD and the formation of RD dimers. We have found this ‘active-like’ conformation of KdpE-RD in structures of KdpE and KdpE-E216A complexed to DNA as well as that of the isolated RD of the non-phosphorylatable KdpE-D52A variant. The active-like conformation of RDs is independent of the phosphorylation state, the crystallization conditions and the crystal contacts. Alternatively, active-like conformation of RDs may be driven by high concentration of proteins in crystals. This conclusion is supported by our studies demonstrating that overexpression of KdpE leads to reporter expression independent of the cognate kinase and of the activation signal, which is changes in K + concentrations. Our results are also consistent with the findings that overexpression of RRs PhoP [44] and UhpA [45] in the absence of a the cognate kinase results in gene transcription. The structure of the KdpE–DNA complex reveals a novel heterodomain interface. In the active-like KdpE–DNA complex structure, the breakdown of symmetry between RDs (two-fold dimers) and DBDs (bound to direct repeats) and the placement of KdpE protomers on one face of the DNA helix implies that a specific set of interactions between RDs and DBDs can occur only between one of the two KdpE molecules in the complex. A unique set of interactions between the α3-loop-β4 of the RD and DBD of KdpE A (compact) subunit is observed. An equivalent set of interactions between the RD and DBD of the extended subunit KdpE B is not possible because α3-loop-β4 of the RD is on the opposite side resulting from the two-fold symmetry of the RD dimers. Speculation of a functional role for the observed RD–DBD interface in KdpE–DNA complex conforms to the idea that molecular surfaces play a significant role in RR-mediated regulation [17] . The potential of the novel RD–DBD interface to influence gene expression was investigated by targeted mutagenesis. Interfacial residues D66 and W70 from RD and R141 and R158 from DBD when substituted with alanine reduce gene expression. A similar alanine substitution of Q69 of the RD results in an altered threshold for activation of gene expression, whereas replacement with large, charged residues, Arg and Glu restores wild-type behaviour ( Fig. 4b ). The data suggests that the distance between the domains may be important to RR-mediated gene expression. Residues D66, Q69 and W70, components of the helix α3 and the loop connecting α3-β4 is a continuation of the polypeptide chain from the active-site residue D52 located on the loop between β3-α3. Helix α3 and the loop connecting α3-β4 are a part of the so-called ‘3445’ face (α3–β5 secondary structure elements), identified as a potential switch region of the RD of NtrC [36] . Activation-induced changes in NtrC included large chemical shifts, displacement of α-helices 3 and 4 and β-strands 4 and 5, register shift and axial rotation of α4 (refs 14 , 16 ). Interestingly, our structure–function studies show residues in the so-called switch region participate in heterodomain interactions to regulate gene expression. In OmpR/PhoB family, active conformation of RD promotes higher affinity DNA interactions leading to a stable complex. In some RRs, RDs in an inactive state interact with DBDs to prevent DNA binding [19] , [20] , [46] , whereas in others, DBDs are free to interact with DNA. Similar to OmpR [25] , KdpE, does not form inhibitory interactions as demonstrated by lack of gene expression by isolated DBD [39] and the relatively tight binding to DNA ( Fig. 1 ). Irrespective of the inhibitory interactions of RD or the lack thereof, activation leads to formation of symmetrical RD-RD dimers. In case of KdpE, the RD-RD dimer buries a larger surface area (795 Å 2 per monomer). Additionally, a unique RD–DBD interface is created along with a DBD–DBD interface in the DNA-bound form of KdpE. Therefore, the overall effect of activation is the formation of multiple interfaces: the intermolecular RD-RD interface; the intramolecular heterodomain RD–DBD interface; and the intermolecular, DBD–DBD interface. Together, the interfaces bury a total of 1,520 Å 2 of surface per KdpE molecule, more than the 1,000 Å 2 required to form stable oligomers and complexes [47] . Disruption of the RD–DBD interface affects transcription ( Fig. 4b ), suggesting interfaces other than the classical RD-RD dimeric interface are necessary to form stable complexes. Such stable RR–DNA complexes are likely to facilitate the assembly of the RNA polymerase at promoters controlled by RRs. Protein purification and characterization KdpE and its variants were overexpressed in E. coli and purified using methods developed for purification of the isolated DBD of KdpE [39] . For electrophoretic mobility shift analysis, the primers with the sequence 5′-CATTTTTATACTTTTTTTACACCCCGCCCG-3′ and its complementary sequence were annealed to produce double-stranded DNA molecules. A volume of 2 μl of DNA at 5 pmoles per μl was mixed with twofold molar concentration of protein in a 10-μl reaction. After 10 min, the mixture was loaded on a 6% acrylamide gel made of TBE buffer (89 mM Tris base, 89 mM boric acid, 2 mM EDTA) [39] . Following electrophoresis, the gels were imaged after staining with ethidium bromide. To analyze the expression of the reporter β-galactosidase, E. coli RH003 cells [(Δ kdpDE , kdpFABC promoter- lacZ + fusion, kdp ABCDE81 , Δ (lac-pro) ara, thi ) were transformed with plasmids carrying KdpD and KdpE genes (except for data shown in Fig. 3b , where KdpD was excluded) and selected on KLM medium (1% KCl, 1% casein hydrolysate, 0.5% yeast extract) supplemented with ampicillin and kanamycin. Cultures were grown to mid-logarithmic phase in minimal medium containing 0.1 mM K + (K0) or 10 mM K + (K10) [39] . Cells were harvested from 1 ml of culture, re-suspended in 1 ml of phosphate-buffered saline containing 5 mM β-mercaptoethanol. SDS and chloroform were added to 0.01% and 0.05% final concentrations, respectively, to lyse the cells. After incubating the lysate at 28 °C for 5 min, 0.2 ml of substrate ortho-nitrophenyl-β-galactoside (4 mg ml −1 ) was added. On the appearance of light yellow colour, the reaction was stopped by adding 0.5 ml of 1 M Na 2 CO 3 and Miller units were calculated (A 420 × min −1 × ml −1 × OD 600 −1 ). SPR analysis The following oligonucleotides were biotin-labelled at the 3′ end: 5′-CATTTTTATACTTTTTTTACACCCCGCCCG-3′ containing the native KdpE-binding sites; and 5′-CATTCCCATACTTTTCCCACACCCCGCCCG-3′ with mutations at the S1 and S2 half-sites that abolish KdpE binding [39] . The biotin-labelled oligonucleotides were annealed to their respective complementary sequences to create double-stranded DNA molecules. The native and mutant DNA molecules were immobilized on Sensor Chip SA (GE Healthcare) at 100 Response Units (RU) on flow channels 2 and 1 using the BiaCore 3000 (GE Healthcare). Purified KdpE-E216A or KdpE in SPR buffer (10 mM HEPES, pH 7.5, 150 mM KCl, 1 mM EDTA, 0.005% Tween 20) was injected at indicated concentrations at a flow rate of 75 μl min −1 . The data collected were processed by removing the values for non-specific binding in channel. Data from three independent replicates were fit to one-site binding model using BIAevaluation software (GE Healthcare) to obtain off-rates. Fluorescence anisotropy assay An oligonucleotide labelled with TAMRA dye via a 5-carbon linker (5′-CATTTTTATACTTTTTTTACACCC-3′) was annealed in SPR buffer to its complementary sequence to produce a double-stranded molecule. KdpE-E216A and KdpE at indicated concentrations were mixed with 5 nM TAMRA-labelled DNA in a 96-well plate. Fluorescence anisotropy was measured at 25 °C in a Spectramax M5 microplate reader (Molecular Devices) with excitation and emission wavelengths set at 530 nm and 590 nm, respectively. Anisotropy data from three independent measurements were fit to a one-site binding model using GraphPad Prism and reported as fractional occupancy. Crystallization and data collection KdpE and KdpE-E216A at a concentration of 200 μM was mixed with 150 μM of 30-bp double-stranded DNA (5′-CATTTTTATACTTTTTTTACACCCCGCCCG-3′) and incubated for 2 h at 25 °C. The protein–DNA mixture was mixed at a 3:1 ratio with well solution (3–5% PEG, 4 K, 0.1 M acetate buffer, pH 5.5, 0.1 M MgCl 2 , 2 mM L -proline) in hanging-drop vapour-diffusion format at 20 °C to obtain crystals. Crystals of KdpE–DNA complex were grown at 12 °C using similar conditions except that the reservoir contained a higher concentration of PEG 4 K (10–15%). The crystals were cryoprotected with 30% PEG 400 in reservoir solution and flash frozen in liquid nitrogen. Diffraction data was collected at the Advanced Photon Source beamline 23-ID-B at GM-CA CAT ( λ =1.0332 Å) and processed using iMosflm 1.0.5 (ref. 48 ). The data collection statistics are shown in Table 1 . Purified RD of KdpE-D52A was dialyzed against 20 mM TRIS (pH 7.5), 100 mM NaCl and concentrated to 15 mg ml −1 . Hexagonal crystals were obtained in 15% PEG, 8 K, 100 mM NaCl, 0.1 mM TRIS (pH 7.2–8.0) using hanging-drop vapour diffusion method at 20 °C in 5–8 days at a protein concentration of 10–12 mg ml −1 . The crystals were soaked (10–20 s) in mother liquor supplemented with 25% glycerol and 0.2 M potassium iodide solution and flash frozen in liquid nitrogen. To obtain anomalous signal of iodine, SAD data set was collected at λ =1.54984 Å using 1° oscillation steps over a total rotation of 360° with an exposure time of 1 s per frame on the 21-IDD beamline at the Advanced Photon Source, Argonne National Laboratory. Data were processed using HKL 2000 and crystallographic data statistics are also shown in Table 1 . Structure determination The molecular replacement method was used to determine the structures of DNA–protein complexes using isolated RD (PDB ID 1ZH4) and DBD (PDB ID 3ZQ7) structures of E. coli KdpE in PHASER 2.4.0 (ref. 49 ), which successfully traced two molecules each of the respective domains in the asymmetric unit. Iterative model building and density modification were carried out in the RESOLVE program integrated into PHENIX AutoBuild wizard [50] . The output model was corrected manually in COOT [51] . The double-stranded DNA was built using PHENIX AutoBuild wizard and manually using the 2Fo-Fc electron density map as guide in COOT [51] . The nucleotide bases in the model were altered manually to match the sequence of the DNA used in crystallization. Structure refinement was carried out using PHENIX and model building and density modification. A model of the biologically relevant complex with two protein molecules occupying DNA half-sites S1 and S2 was generated. Water molecules were also added by manual inspection of 2Fo-Fc electron density map. The final refined model had crystallographic R factor and R free values that were within the range of average values for structures refined at these resolutions [52] . The refinement statistics are reported in Table 1 . The following residues in the linker regions between RD and DBD could not be modelled due to poor electron density: residues 121–123 in Chain A and residues 121–122 in Chain B in KdpE-E216A–DNA complex structure; residues 120–123 from Chain A in KdpE–DNA complex structure. In addition, out of the 30-bp of DNA in the complex, only 24 bp could be modelled due to the poor electron density in the KdpE–DNA complex structure. The structures were validated using comprehensive validation tools in PHENIX [50] , [53] . In KdpE-E216A–DNA complex structure, 96.13% residues are in Ramachandran favored region, whereas 3.64% residues are in allowed region. In KdpE–DNA complex structure, 95.93% residues are in Ramachandran favored region, whereas 4.075% residues are in allowed region. r.m.s.d. ( Supplementary Table 1 ) were calculated using SSM program [54] . Graphics were generated using Chimera 1.6.0 (ref. 55 ) and PyMOL ( http://www.pymol.org ). Diffraction data from a single crystal of RD of KdpE-D52A were processed with HKL 2000 (ref. 56 ) and crystallographic data statistics are shown in Table 1 . The crystals belong to space group P3121 with three protein molecules per asymmetric unit. Substructure solution, phasing and density modification and partial model building was performed using PHENIX AutoSol and AutoBuild wizard. The overall anomalous signal-to-noise ratio is 2.3. A total of 35 iodine sites were located with the Bayesian estimate of map CC and figure of merits of 0.52 and 0.38, respectively. Iterative model building and refinement was performed in COOT and PHENIX. The structures were validated using comprehensive validation tools in PHENIX [50] , [53] . Accession codes : Structure factors and atomic coordinates have been deposited in the Protein Data Bank under accession codes 4KFC and 4KNY for KdpE-E216A–DNA and KdpE–DNA complexes respectively, and 4L85 for KdpE-D52A. How to cite this article: Narayanan, A. et al. An asymmetric heterodomain interface stabilizes a response regulator–DNA complex. Nat. Commun. 5:3282 doi: 10.1038/ncomms4282 (2014).